A toggle switch controls the low pH-triggered rearrangement and maturation of the dengue virus envelope proteins Immature dengue virus particles undergo a dramatic conformational change upon exposure to the acidic environment of the late secretory pathway. The interactions of the E fusion proteins and prM chaperone proteins on the virus envelope are reorganized to permit prM processing by a host protease, furin, thus priming virus for fusion and infection. Here we identify a pH-dependent toggle switch that controls this key conformational change during virus maturation. Our data show that the M region of prM interacts with E at neutral pH but is released at acidic pH, while the pr region interacts with E at acidic pH but is released at neutral pH. Alanine substitution of the conserved residue H98 in prM disrupts the switch by inhibiting dissociation of M from E at low pH, resulting in impaired prM processing and decreased virus infectivity. Thus, release of M–E interaction at low pH promotes formation of a furin-accessible intermediate. Dengue virus (DENV) is a significant human pathogen that is transmitted by mosquitoes and produces a wide range of clinical manifestations ranging from acute febrile illness to life-threatening dengue haemorrhagic fever and dengue shock syndrome (reviewed in ref. 1 , 2 , 3 ). DENV is now endemic in more than 100 countries, with more than a third of the world’s population at risk of infection. Recent analysis suggests that annually there are ~390 million DENV infections worldwide, and about 96 million cases of apparent disease [4] . In spite of this disease burden, there are as yet no licensed DENV vaccines or antiviral therapies. DENV has four well-characterized serotypes (DENV1–4) and belongs to the flaviviruses, a genus of small spherical enveloped plus-sense RNA viruses (reviewed in refs 5 , 6 ). DENV particles contain a nucleocapsid core composed of the RNA genome packaged by the capsid protein. This core is enveloped by the virus membrane, which is covered by a highly organized lattice of the E and M envelope proteins. DENV enters cells by receptor-mediated endocytosis [7] , [8] . The low pH environment of the late endosome triggers virus–membrane fusion, delivering the viral genome into the cytoplasm for replication [7] , [8] , [9] . Progeny virus particles bud into the endoplasmic reticulum (ER) and are released by transit through the cellular secretory pathway [5] . Both virus–receptor binding and virus–membrane fusion are mediated by E, an elongated protein composed of three β-sheet-rich domains with the membrane anchor on one side and a hydrophobic fusion loop at the membrane distal tip [10] , [11] , [12] , [13] , [14] , [15] . In the mature virus particle, E is organized in homodimers with the fusion loop concealed within the dimer interface [16] . During virus entry, low pH triggers the dissociation of the E dimer, insertion of the fusion loop into the endosome membrane and refolding to a trimeric E hairpin to drive membrane fusion [17] , [18] . The DENV structural proteins capsid, prM, and E are translated as part of a polyprotein that also encodes the nonstructural proteins [5] . The envelope protein prM is a chaperone that assists in E folding and is composed of an N-terminal globular pr region (residues 1–91) and the M ectodomain (92–130) connecting to the membrane anchor [19] . prM and E dimerize within the ER [20] and organize into spike-like trimers of (prM+E) on the nascent virus particle [21] . However, this immature virus is noninfectious and the E fusion loop is covered by the pr region [19] , [22] , [23] . During transport through the secretory pathway, the virus is exposed to the mildly acidic environment of the Golgi, trans-Golgi network and secretory vesicles [24] . Low pH triggers a striking rearrangement of the spiky immature virus into a relatively smooth-surfaced particle in which dimers of (prM+E) are oriented tangential to the virus membrane [19] , [22] , [23] . This rearrangement makes prM accessible to cleavage by the cellular protease furin, producing the mature M protein and the pr peptide [23] , [25] . At low pH, pr remains bound to the E protein tip and prevents premature virus fusion and E protein membrane insertion [22] , [26] . In the final step of maturation, secretion of the virus into the neutral pH extracellular milieu allows the release of pr to produce infectious mature virus containing E and M [19] , [22] , [23] , [26] . Furin processing of prM is typically incomplete, but such partially mature viruses are infectious [27] , [28] , [29] . Complete processing of prM can be driven by furin overexpression [27] , while the fully immature noninfectious virus can be produced by treatment of infected cells with NH 4 Cl, which neutralizes the low pH in the secretory pathway and prevents particle rearrangement [25] , [30] , [31] , [32] . The low pH-triggered conformational rearrangement of the prM and E proteins is thus critical for DENV maturation and infectivity, but its mechanism is as yet unclear. What might control this key conformational change? Rearrangement of the immature virus is blocked by high concentrations of Fab antibody against pr [33] , suggesting that the pr–E interaction could be involved. While the structure of the prM–E dimer does not show significant differences in the pr–E interface at neutral versus low pH [19] , the arrangement in virus could differ [34] . The prM–E dimer structure does not resolve the M ectodomain [19] , but fitting of the structure into cryo-EM reconstructions of mature and immature virus suggests that M rearranges during the conformational change [19] . Recent cryo-EM reconstructions of immature and mature DENV1 suggest that the M N-terminal region interacts with E domain II in both the mature and immature particles [34] . In vitro , a purified peptide containing residues 111–131 of M binds to both E protein and liposomes at low pH, suggesting a dual low pH-dependent interaction of this M region with E and the virus membrane that could trigger surface protein rearrangement [35] . A recent 3.5 Å reconstruction of mature DENV2 led to a model in which the unfolded region of pr (residues 81–91) in prM acts as a drawstring at low pH, pulling on the pr globular domain that covers the E tip to trigger the conformational change [36] . Indeed, such a drawstring model was proposed in the original structural study of the prM–E dimer [19] . In addition, significant movements of the M protein stem and transmembrane (TM) regions occur during particle maturation, and could potentially play a role [15] , [34] . However, while a variety of models have been proposed for the DENV maturation pathway, experimental validation has lagged behind, and the differences between the models remain unresolved. Here we address the mechanism of low pH-triggered DENV rearrangement, a critical step in the pathway of virus maturation. Our data indicate that the M region of prM binds E at neutral pH and is released at acidic pH. This pH-dependent switch requires a conserved histidine residue at position 98 of prM, and the absence of H98 strongly impairs prM processing and DENV infection. Our data thus identify a novel mechanism that controls the production of a furin-accessible intermediate in the virus maturation pathway. pH-dependent interaction of M region with E protein To probe for interactions between the DENV prM and E proteins, we transfected 293T cells with a plasmid encoding the DENV1 prME polyprotein, lysed the cells in buffer at pH 6.0 or pH 7.4 and assayed for prM–E binding by immunoprecipitation using a monoclonal antibody (mAb) against prM ( Fig. 1 ). The wild-type (WT) E protein was observed to co-immunoprecipitate (co-IP) with prM in both neutral and low pH buffers. Given that the pr peptide binds to the E protein at low but not neutral pH [22] , [26] , this result suggested that the interaction of prM and E at neutral pH was mediated by the M region. To more specifically measure the interaction of the M region with E, we introduced an alanine substitution at residue H244 in the E protein. This histidine lies in the pr–E interface interacting with pr D64 and D65, and the E H244A substitution was previously demonstrated to inhibit pr–E binding [26] . Co-IP assays of lysates of prM–E H244A expressing cells indicated that the M region bound the H244A E protein at pH 7.4 but not at pH 6.0. Co-IP assays using a mAb against the E protein produced similar results ( Supplementary Fig. 1 ), indicating that the observed binding was independent of the protein targeted by the mAb. Our results thus suggest that the pr and M regions both interact with the E protein but show inverse pH dependence, with M binding E at neutral pH and pr binding E at low pH. 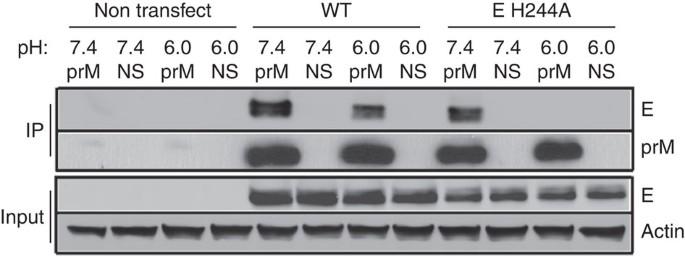Figure 1: The M region of DENV prM protein binds E protein at neutral pH. 293T cells were transfected as indicated with plasmids encoding the WT or mutant prME (that is, ‘E H244A’). Two days post transfection, the cells were lysed in buffers at the indicated pH. Aliquots of the lysates were immunoprecipitated at the indicated pH with anti-prM mAb 38.1 (prM) or a non-specific mAb (NS) and analysed by SDS–PAGE and western blot to detect prM or E. Expression levels in the lysates were evaluated by western blot analysis (input). The data are a representative example of five independent experiments. Full scans of the blots are inSupplementary Fig. 4. Figure 1: The M region of DENV prM protein binds E protein at neutral pH. 293T cells were transfected as indicated with plasmids encoding the WT or mutant prME (that is, ‘E H244A’). Two days post transfection, the cells were lysed in buffers at the indicated pH. Aliquots of the lysates were immunoprecipitated at the indicated pH with anti-prM mAb 38.1 (prM) or a non-specific mAb (NS) and analysed by SDS–PAGE and western blot to detect prM or E. Expression levels in the lysates were evaluated by western blot analysis (input). The data are a representative example of five independent experiments. Full scans of the blots are in Supplementary Fig. 4 . Full size image Role of prM H98 in E binding Given these results, we hypothesized that there might be a switch from M–E to pr–E binding during transit of immature DENV from the neutral pH of the ER to the low pH of the late secretory pathway. Such a switch could contribute to the known low pH-triggered rearrangement of the virus particle and thus facilitate DENV maturation. Sequence comparisons showed that a histidine at position 98 in the M region is strictly conserved among all flaviviruses ( Fig. 2a ), and the pKa of histidine (~6–6.5) [37] , [38] as well as the prM–E structural studies [19] suggested its possible involvement in the pH-dependent binding we observed between the M region and E protein. To test this, we substituted alanine for prM H98 in the WT and E H244A prME expression constructs. Co-IP analysis showed that, like the WT prM ( Fig. 2b , lanes 1–4), H98A prM bound E at both pH 6.0 and pH 7.4 ( Fig. 2b , lanes 5–8). While the WT prM showed no co-IP at low pH when tested with E protein containing the H244A substitution ( Fig. 2b , lanes 9–12), the H98A prM showed efficient co-IP of H244A E protein at both neutral and low pH ( Fig. 2b , lanes 13–16). Thus, the H98A mutation inhibited the low pH-induced release of the M region-E interaction. Together, these results suggest a model in which prM–E association toggles between M–E binding at neutral pH versus pr–E binding at low pH ( Fig. 2c ). 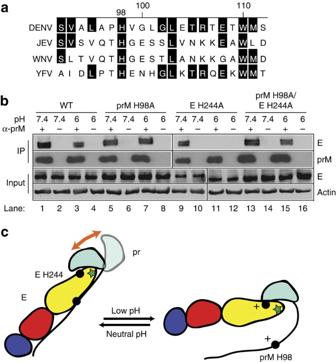Figure 2: DENV M H98 is a key residue in M–E binding. (a) Sequence comparison of M protein residues 92–112 (DENV numbering) from four representative flaviviruses: DENV1 western Pacific (DENV), Japanese encephalitis virus (JEV Nakayama strain, JEV), West Nile virus (WNV NY99 strain, WNV) and Yellow Fever virus (YFV 17D strain, YFV). The alignment was generated by ClustalW and residues conserved versus the DENV sequence are highlighted in black. (b) The prM H98A mutation inhibits prM–E dissociation at acidic pH. WT or H98A prM was assayed for binding with WT or H244A E protein by co-IP as described inFig. 1. α-prM indicates mAb 38.1. The data are a representative example from one of three independent experiments. Full scans of the blots are inSupplementary Fig. 4. (c) Model for the pH-dependent switch of pr–E and M–E interaction. E protein DI, DII and DIII are coloured in red, yellow and blue, respectively, with the green star indicating the fusion loop. In the prM protein, pr is coloured in cyan and the M ectodomain is shown as a black line. Residues E H244 and prM H98 are indicated in the model as solid circles, with a +sign to indicate their protonation at low pH. The orange arrow in the left panel indicates the relatively loose interaction of the pr region with E at neutral pH. Figure 2: DENV M H98 is a key residue in M–E binding. ( a ) Sequence comparison of M protein residues 92–112 (DENV numbering) from four representative flaviviruses: DENV1 western Pacific (DENV), Japanese encephalitis virus (JEV Nakayama strain, JEV), West Nile virus (WNV NY99 strain, WNV) and Yellow Fever virus (YFV 17D strain, YFV). The alignment was generated by ClustalW and residues conserved versus the DENV sequence are highlighted in black. ( b ) The prM H98A mutation inhibits prM–E dissociation at acidic pH. WT or H98A prM was assayed for binding with WT or H244A E protein by co-IP as described in Fig. 1 . α-prM indicates mAb 38.1. The data are a representative example from one of three independent experiments. Full scans of the blots are in Supplementary Fig. 4 . ( c ) Model for the pH-dependent switch of pr–E and M–E interaction. E protein DI, DII and DIII are coloured in red, yellow and blue, respectively, with the green star indicating the fusion loop. In the prM protein, pr is coloured in cyan and the M ectodomain is shown as a black line. Residues E H244 and prM H98 are indicated in the model as solid circles, with a +sign to indicate their protonation at low pH. The orange arrow in the left panel indicates the relatively loose interaction of the pr region with E at neutral pH. Full size image The prM H98A mutation inhibits DENV1 VLP prM processing The binding results above suggested that the prM H98A mutation might allow us to determine the connection between M region–E interaction and DENV maturation. We hypothesized that interference with this interaction would block the conformational rearrangement of the virus at low pH, inhibiting prM maturation. We tested maturation using the virus-like particles (VLP) produced by cells expressing prME, a system that has been used extensively to study flavivirus assembly, maturation, secretion and membrane fusion [26] , [39] , [40] , [41] . The WT- and prM H98A mutant-transfected cells both showed efficient prM and E expression and had similar secretion of VLPs ( Fig. 3a ). However, processing of prM was markedly less efficient in cells expressing prME proteins with the prM H98A mutation, with a ratio of prM/(M+prM) about 2.7 times higher than that of the WT. 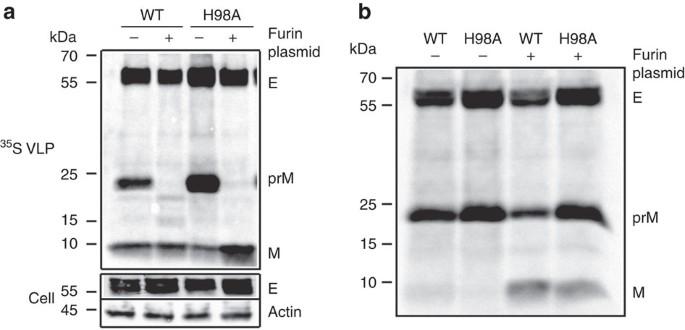Figure 3: prM H98A mutation inhibits prM processing. (a) The prM H98A mutation decreases DENV prM processing. 293T cells were transfected with plasmids encoding WT or mutant DENV1 prME (H98A) with or without co-transfection with a plasmid encoding furin. After 12 h, cells were radiolabelled for 36 h with35S-methionine/cysteine. VLPs were pelleted and analysed by SDS–PAGE and phosphorimaging (‘35S VLP’). The cell lysates were analysed by SDS–PAGE and western blot using mAbs to E protein and β-actin (‘cell’). Quantitative western blot analysis showed that E protein expression in the mutant was ~1.8–2.2-fold that of the WT and efficiency of H98A VLP secretion ranged from 0.8–1.1-fold that of WT (n=3). (b) Furin overexpression drives prM processing at neutral pH. WT and mutant VLPs were produced and analysed as inFig. 3aexcept that radiolabelling was performed in the presence of 20 mM NH4Cl to neutralize exocytic pH. Data inaandbare representative examples of three independent experiments. Full scans of the phorphorimages and blots are inSupplementary Fig. 4. Figure 3: prM H98A mutation inhibits prM processing. ( a ) The prM H98A mutation decreases DENV prM processing. 293T cells were transfected with plasmids encoding WT or mutant DENV1 prME (H98A) with or without co-transfection with a plasmid encoding furin. After 12 h, cells were radiolabelled for 36 h with 35 S-methionine/cysteine. VLPs were pelleted and analysed by SDS–PAGE and phosphorimaging (‘ 35 S VLP’). The cell lysates were analysed by SDS–PAGE and western blot using mAbs to E protein and β-actin (‘cell’). Quantitative western blot analysis showed that E protein expression in the mutant was ~1.8–2.2-fold that of the WT and efficiency of H98A VLP secretion ranged from 0.8–1.1-fold that of WT ( n =3). ( b ) Furin overexpression drives prM processing at neutral pH. WT and mutant VLPs were produced and analysed as in Fig. 3a except that radiolabelling was performed in the presence of 20 mM NH 4 Cl to neutralize exocytic pH. Data in a and b are representative examples of three independent experiments. Full scans of the phorphorimages and blots are in Supplementary Fig. 4 . Full size image Processing of the WT flavivirus prM is incomplete and can be rescued by overexpression of the furin protease [42] . Co-transfection with a plasmid encoding human furin resulted in complete processing of both the WT and the prM H98A-mutant prM proteins ( Fig. 3a ). Given our hypothesis that the prM H98A mutation blocked particle rearrangement at low pH, the complete furin processing of the mutant was puzzling. We therefore tested if the high levels of furin expression made processing relatively independent of virus conformation. VLPs were produced in cells treated with NH 4 Cl ( Fig. 3b ), a treatment known to neutralize the pH in the secretory pathway [24] , [26] . The enzymatic activity of mature furin has a neutral pH optimum [23] , [25] , and its autocatalytic maturational process is also relatively efficient at neutral pH [43] . While NH 4 Cl treatment inhibited maturation of both WT and mutant prM as expected, overexpression of furin increased the processing of both WT and mutant prM proteins, resulting in prM/(M+prM) ratios similar to those of WT under control conditions. Thus, furin overexpression promotes processing even under conditions known to trap the virus in the neutral pH, ‘spiky’ form. prM H98A decreases DENV maturation and infectivity The VLP system does not package the viral genome and the particles are smaller than those of authentic flavivirus [40] , [41] . To test the effect of prM H98A on virus infectivity, we therefore used a recombinant virus particle (RVP) system that encapsidates a green fluorescent protein (GFP) reporter and supports single-cycle infection [44] . The WT and prM H98A viruses showed similar levels of viral protein expression and virus particle production ( Fig. 4a ). As observed in the VLP system, the prM H98A mutation inhibited prM processing, resulting in a prM/(M+prM) ratio ~2.1 times higher than the WT. The prM H98A mutation reduced the RVP titre by ~ 2 logs compared with WT ( Fig. 4b ). Furin overexpression rescued both prM H98A prM processing ( Fig. 4a ) and prM H98A virus infectivity ( Fig. 4b ) to levels comparable with those of WT. 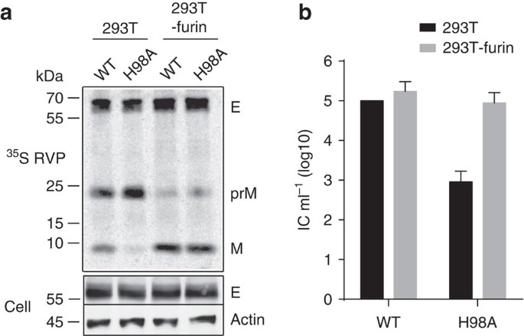Figure 4: prM H98A inhibits DENV RVP maturation and infection. (a) prM H98A inhibits prM processing. RVPs were produced in control or furin-overexpressing 293T cells by co-transfection of plasmids encoding the WT or mutant DENV1 WP structural proteins and a WNV replicon plasmid encoding the nonstructural proteins plus a GFP reporter. Starting at 12 h post transfection, cells were radiolabelled at 29 °C for 36 h. RVPs and cell lysate samples were harvested and analysed as inFig. 3a. Data are a representative example of three independent experiments. Quantitation of western blots and35S-labelling showed that E protein expression in mutant-infected cells was 1.2–1.3-fold that of the WT, and efficiency of RVP secretion was 0.8–0.9-fold that of WT (n=2). Full scans of the phorphorimages and blots are inSupplementary Fig. 4. (b) prM H98A inhibits DENV RVP infectivity and is rescued by furin overexpression. WT and mutant RVPs were produced in control or furin-overexpressing 293T cells as in 4a but without radiolabelling. The resultant RVPs were titered on Vero cells. Data in panel 4b are the mean and s.d. of four independent experiments, with WT titers produced in 293T cells normalized to 105infectious units ml−1. Figure 4: prM H98A inhibits DENV RVP maturation and infection. ( a ) prM H98A inhibits prM processing. RVPs were produced in control or furin-overexpressing 293T cells by co-transfection of plasmids encoding the WT or mutant DENV1 WP structural proteins and a WNV replicon plasmid encoding the nonstructural proteins plus a GFP reporter. Starting at 12 h post transfection, cells were radiolabelled at 29 °C for 36 h. RVPs and cell lysate samples were harvested and analysed as in Fig. 3a . Data are a representative example of three independent experiments. Quantitation of western blots and 35 S-labelling showed that E protein expression in mutant-infected cells was 1.2–1.3-fold that of the WT, and efficiency of RVP secretion was 0.8–0.9-fold that of WT ( n =2). Full scans of the phorphorimages and blots are in Supplementary Fig. 4 . ( b ) prM H98A inhibits DENV RVP infectivity and is rescued by furin overexpression. WT and mutant RVPs were produced in control or furin-overexpressing 293T cells as in 4a but without radiolabelling. The resultant RVPs were titered on Vero cells. Data in panel 4b are the mean and s.d. of four independent experiments, with WT titers produced in 293T cells normalized to 10 5 infectious units ml −1 . Full size image Rescue of the pH switch by second-site revertants of prM H98A Using a DENV1 infectious clone [45] , we demonstrated that the prM H98A mutation inhibited virus infection ( Fig. 5a ) and viral prM processing ( Fig. 5b ) without affecting virus particle production. We used the mutant virus-infected cells to select for rescue mutations that might define features of the prM–E interaction. As shown in Table 1 , each independent revertant contained one or two second-site mutations in prM (E104V) and/or E (E62K, V130A, E202K). We tested a subset of these mutations by expressing each in RVPs containing prM H98A ( Fig. 6 ). None of the mutations significantly affected protein expression or RVP secretion ( Fig. 6b ). When produced in 293T cells, the ratio of prM/(M+prM) of the H98A RVP was about twice that of the WT and was rescued to the WT level by both the E E62K and prM E104V mutations ( Fig. 6b ). Both E E62K and prM E104V also significantly increased (~1.6 log) the infectivity of prM H98a RVP ( Fig. 6a ). In contrast, the E E202K mutation produced no significant rescue of prM H98A processing (prM/E ratio ~2.1 times that of WT) and caused only a minor increase in prM H98A titre. All of the RVPs produced in 293T-furin cells showed similar titres of ~10 5 IC ml −1 and nearly complete processing of prM ( Fig. 6a,b ). These results suggest that the dissociation of M from E normally mediated by H98 protonation could be triggered by a shift towards a more positive net charge at sites on either M or E ( Table 1 ). To test this directly, the prM E104V mutation was introduced into the expression plasmid encoding DENV1 prM H98A+E H244A, and prM–E interaction tested by co-IP ( Fig. 7 ). prM H98A stabilized the interaction between prM and E H244A at pH 6.0, and this stabilization at low pH was reversed by the prM E104V mutation, but was unchanged at neutral pH ( Fig. 7 ). Thus the second-site revertants coordinately affected prM–E binding, prM processing and virus infectivity. 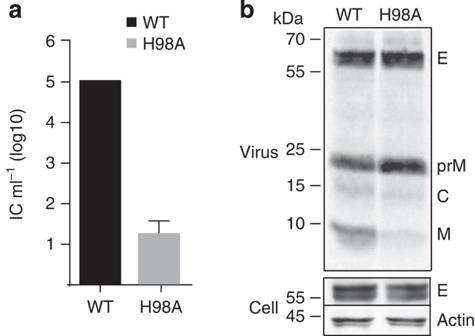Figure 5: prM H98A mutation inhibits DENV maturation and infection. (a) Test of infectivity. RNAs derived from the WT and prM H98A DENV1 WP infectious clones were electroporated into 293T cells. Progeny virus was collected 4 days post electroporation and titered on BHK-21 cells. Data are the mean and s.d. of three independent experiments, with WT titres normalized to 105IC ml−1. (b) Test of prM processing. RNAs derived from the WT and prM H98A DENV1 WP infectious clones were electroporated into 293T cells. Cells were radiolabelled with35S methione/cysteine for 4 days at 29 °C. Virus in the labelling medium was pelleted by ultracentrifugation, immunoprecipitated with mouse anti-DENV2 serum and analysed by SDS–PAGE and phosphorimaging (‘virus’). The cell lysates were analysed by SDS–PAGE and western blot using mAbs to E protein and β-actin (‘cell’). Positions of molecular weight markers are shown on the left. Data are a representative example of three independent experiments. Full scans of the phorphorimages and blots are inSupplementary Fig. 4. Figure 5: prM H98A mutation inhibits DENV maturation and infection. ( a ) Test of infectivity. RNAs derived from the WT and prM H98A DENV1 WP infectious clones were electroporated into 293T cells. Progeny virus was collected 4 days post electroporation and titered on BHK-21 cells. Data are the mean and s.d. of three independent experiments, with WT titres normalized to 10 5 IC ml −1 . ( b ) Test of prM processing. RNAs derived from the WT and prM H98A DENV1 WP infectious clones were electroporated into 293T cells. Cells were radiolabelled with 35 S methione/cysteine for 4 days at 29 °C. Virus in the labelling medium was pelleted by ultracentrifugation, immunoprecipitated with mouse anti-DENV2 serum and analysed by SDS–PAGE and phosphorimaging (‘virus’). The cell lysates were analysed by SDS–PAGE and western blot using mAbs to E protein and β-actin (‘cell’). Positions of molecular weight markers are shown on the left. Data are a representative example of three independent experiments. Full scans of the phorphorimages and blots are in Supplementary Fig. 4 . Full size image Table 1 Second-site revertants of prM H98A*. 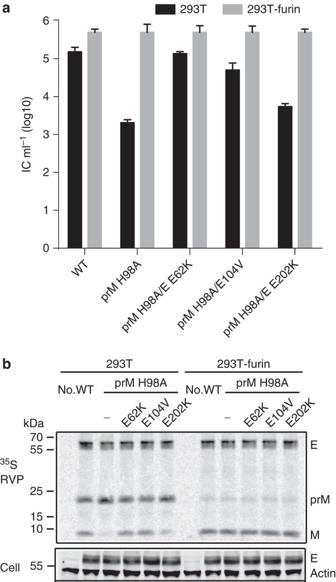Figure 6: Second-site mutations in prM and E rescue the maturation of prM H98A DENV. (a) Second-site mutations rescue the infectivity of prM H98A virus. Individual mutations were introduced into the DENV1 prM H98A structural proteins, and RVPs were produced and titered as forFig. 4a. Titres were normalized to that of the WT from 293T-furin cells. Data shown are the mean±s.d. of three independent experiments. (b) Second-site mutations rescue the maturation of prM H98A RVPs. Radiolabelled WT and mutant RVPs were produced and analysed as forFig. 4b. Note that E104V indicates a mutation in prM (seeTable 1). ‘No.’ indicates uninfected cells. Data are a representative example of two independent experiments. Quantitation of western blots and35S-labelling showed that E protein expression in mutant-infected cells was 0.8–1.4-fold that of the WT, and efficiency of RVP secretion ranged from 0.6–1.2-fold that of WT (n=2). Full scans of the phorphorimages and blots are inSupplementary Fig. 4. Full size table Figure 6: Second-site mutations in prM and E rescue the maturation of prM H98A DENV. ( a ) Second-site mutations rescue the infectivity of prM H98A virus. Individual mutations were introduced into the DENV1 prM H98A structural proteins, and RVPs were produced and titered as for Fig. 4a . Titres were normalized to that of the WT from 293T-furin cells. Data shown are the mean±s.d. of three independent experiments. ( b ) Second-site mutations rescue the maturation of prM H98A RVPs. Radiolabelled WT and mutant RVPs were produced and analysed as for Fig. 4b . Note that E104V indicates a mutation in prM (see Table 1 ). ‘No.’ indicates uninfected cells. Data are a representative example of two independent experiments. Quantitation of western blots and 35 S-labelling showed that E protein expression in mutant-infected cells was 0.8–1.4-fold that of the WT, and efficiency of RVP secretion ranged from 0.6–1.2-fold that of WT ( n =2). Full scans of the phorphorimages and blots are in Supplementary Fig. 4 . 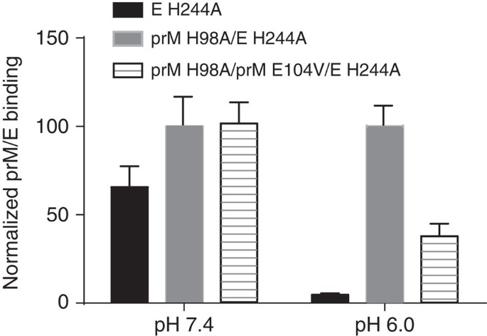Figure 7: The revertant mutation prM E104V rescues the phenotype of M region-E dissociation at low pH. 293T cells were transfected with plasmids encoding prME proteins containing the indicated mutations. The prM/E interaction at the indicated pH was quantitated by co-IP using mAb 38.1 as inFig. 1. The prM E104V revertant mutation decreases prM H98A binding to E H244A at low pH. Data shown are the mean±s.d. of three independent experiments, with the co-IP normalized to that obtained for prM H98A/E H244A for each pH. The average co-IP for prM H98A/E H244A at pH 6.0 was 33% of that at pH 7.0. Full size image Figure 7: The revertant mutation prM E104V rescues the phenotype of M region-E dissociation at low pH. 293T cells were transfected with plasmids encoding prME proteins containing the indicated mutations. The prM/E interaction at the indicated pH was quantitated by co-IP using mAb 38.1 as in Fig. 1 . The prM E104V revertant mutation decreases prM H98A binding to E H244A at low pH. Data shown are the mean±s.d. of three independent experiments, with the co-IP normalized to that obtained for prM H98A/E H244A for each pH. The average co-IP for prM H98A/E H244A at pH 6.0 was 33% of that at pH 7.0. Full size image Role of M H98 in the pH dependence of DENV membrane fusion Structural studies of mature DENV localized M H98 within the ‘hole’ between the two E proteins in the E homodimer [36] . Note that this report uses the mature M numbering, H7. The authors proposed a ‘latch’ model in which uncharged M protein would restrain the E dimers until exposure to low pH protonates M H98 and adjacent E histidine residues, leading to M–E repulsion, release of the latch and fusion. Our results ( Fig. 4b ) indicated that the prM H98A substitution had no significant effect on the infectivity of mature DENV RVPs. However, maximal fusion of DENV occurs at ~pH 6.2 or below [46] , while the pH of endosomes ranges from ~6.5 to 5.5 (ref. 47) [47] . Thus, an acidic shift in the pH dependence of DENV fusion might not cause a deleterious effect on virus growth in cell culture. To specifically test the role of M H98 in the low pH-triggered fusion reaction, we produced mature WT or prM H98A RVP, bound them to BHK cells and triggered their fusion with the plasma membrane by a 1 min low pH pulse. The WT and prM H98A-mutant viruses showed very similar pH dependence of fusion, with maximal fusion of both at ~pH 6.25 ( Fig. 8 ). Thus, our data strongly support a key role of prM H98 in the low pH-triggered rearrangement and maturation of the immature DENV particle but not in the fusion reaction of the mature virus. 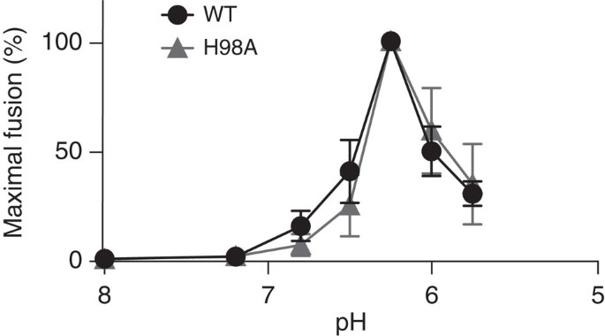Figure 8: The prM H98A mutation does not affect the pH dependence of DENV fusion. Mature WT and prM H98A RVPs were produced in 293T-furin cells as inFig. 4a. Mature RVPs were bound to BHK-21 cells on ice for 90 min and then treated at the indicated pH at 37 °C for 1 min to trigger virus–plasma membrane fusion. Cells infected by RVP fusion were quantitated by scoring GFP-positive cells, and the results are shown as percentage of the maximal fusion for each RVP. Data shown are the mean±s.d. of three independent experiments. Figure 8: The prM H98A mutation does not affect the pH dependence of DENV fusion. Mature WT and prM H98A RVPs were produced in 293T-furin cells as in Fig. 4a . Mature RVPs were bound to BHK-21 cells on ice for 90 min and then treated at the indicated pH at 37 °C for 1 min to trigger virus–plasma membrane fusion. Cells infected by RVP fusion were quantitated by scoring GFP-positive cells, and the results are shown as percentage of the maximal fusion for each RVP. Data shown are the mean±s.d. of three independent experiments. Full size image The low pH-triggered rearrangement of the DENV envelope proteins is critical for virus maturation and infectivity, but its regulation and mechanism were unclear. Our data demonstrated that prM acts as a pH-sensitive switch, toggling from an initial M–E interaction to a pr–E interaction during transport through the pH gradient of the secretory pathway. The conserved prM H98 was a key residue in the switch, required for the release of the M region from E at low pH and thus promoting prM processing and virus infectivity. Considered in the context of the structures of the immature virus and the prM–E dimer [19] , [22] , [23] , our data suggest a model for the molecular mechanism of DENV maturation ( Supplementary Fig. 2 ). In the neutral pH environment of the ER, the strong interaction of the M region of prM with E prevents the formation of E homodimers in the nascent immature virus. The pr region is stabilized at the E tip by its connection to M. The prM–E heterodimers assemble into the trimeric immature spike complex. While a number of interactions probably act to drive spike trimer formation, it may be promoted by pr–pr contacts at the trimer tip [19] , [33] , [34] . Virus particles then bud and transit through the secretory pathway. Exposure to the low pH in the late Golgi/TGN causes protonation of the key histidine residues prM H98 and E H244, thus producing electrostatic repulsion between the M region and E while increasing the binding of the pr region to E. Together, these interactions promote conversion of the spiky trimer to the smooth dimer conformation to expose the furin cleavage site and allow virus maturation. In contrast to our results, previous studies found that a peptide containing residues 111–131 of the DENV M ectodomain had higher binding to both the E protein ectodomain and liposomes at low pH versus neutral pH [35] . The efficiency of peptide binding in these studies and its relationship to the behaviour of the complete protein are unknown. In addition, the E protein ectodomain used in these experiments was produced in the absence of the prM chaperone, which may affect the E conformation. Also, in contrast, studies of the flavivirus Japanese encephalitis virus found that alanine substitution of prM H99 (JEV numbering) inhibits prM–E interaction in a co-IP assay and prevents VLP production [48] . However, these results are based on prM and E proteins produced in trans using baculovirus expression, and the effects of pH on binding were not tested. Together, our results with VLP, RVP and infectious DENV demonstrate that a prM H98A mutation acts to block the low pH-triggered release of the M region from E, a pH-dependent switch that controls prM–E interaction and virus maturation. Our findings suggest a mechanism involving electrostatic repulsion between protonated prM H98 and hydrophobic or positively charged residues on the E protein. The prM H98A mutation disrupted this half of the pH-dependent toggle switch by inhibiting M region dissociation from the E protein. Analysis of revertants identified second-site mutations on prM and E that partially rescue the maturation and infectivity of the prM H98A mutant. The rescue mutations tended to increase the net positive charge in the M region or in E protein, and a direct test of one (prM E104V) showed that it promoted the release of the prM H98A region from E protein at low pH. Thus, our evidence suggests that the revertant mutations function by decreasing the binding affinity between M H98A and E protein at low pH. This may then allow the other half of the toggle switch, the protonation of E H244, to at least partially trigger the conformation change. The H98A rescue mutations are not located in the M–E interface displayed in the immature DENV1 cryo-EM structure [34] . However, only part of the M ectodomain density is reported to be continuous in this reconstruction. The fitting is based on the DENV2 prM–E hybrid protein structure [19] in which the prM and E ectodomains are connected by an 8-residue linker whose length is ~26 Å as determined in other structural studies [49] . In contrast, the observed distance between the C-terminus of the prM ectodomain and the N terminus of E in the immature DENV1 cryo-EM reconstruction is ~35 Å, suggesting that the relatively short linker length in the hybrid protein may affect the positioning of the M region in the hybrid protein fitting. It thus seems plausible that the rescue mutations at E protein positions 62, 130 and 202 identify sites within the M–E interface in the immature virus particle ( Supplementary Fig. 3 ). A recent cryo-EM reconstruction of mature DENV2 shows that the processed M ectodomain contains an extended N-terminal loop (residues 92–111) that lies beneath the E homodimer and interacts with the side of E through hydrophobic contacts [36] . This region of M was suggested to act as a latch that stabilizes the E dimer at neutral pH and would be released by protonation of M H98 and E H209 at low pH [36] , [50] . Our results demonstrated that alanine substitution of M H98 had no detectable effect on the infectivity or pH threshold of mature RVPs. Mutagenesis of H209 in West Nile virus E protein (214 in WNV numbering) produced only very minor effects on virus infectivity [42] . While our data strongly support a role for prM H98 in the low pH-dependent pathway of virus maturation, once mature virus was produced H98 did not play an important role in virus infectivity or fusion. If M does act as a latch, other residues may be more important in its stability and regulation. The rearrangement of the DENV envelope proteins from the spiky trimer to the smooth dimer conformation is a complex and dynamic process involving movements not only of the prM and E ectodomains but also of their transmembrane domains [19] , [34] . An important approach to the study of maturation is the characterization of conformational intermediates in the pathway. Intermediates in DENV maturation have been captured by strategies including antibodies, mutagenesis or pH alterations (for example, refs 22 , 23 , 29 , 33 ). Our results suggest that the prM H98A mutant captures a conformational intermediate generated during transit through the low pH of the secretory pathway. Because furin cleavage is relatively inefficient, WT DENV is normally composed of both prM and M, but can be fully processed by furin overexpression (as shown here and in ref. 27 ). The prM H98A mutant is more resistant to furin cleavage than the WT virus, suggesting that at low pH, the conformation of prM H98A virus differs from that of a smooth immature WT virus ( Supplementary Fig. 2 ). However, our results also suggest that the prM H98A virus is not in the fully immature spiky trimer conformation. WT virus trapped in this spiky conformation by NH 4 Cl treatment was highly resistant to furin processing, and even furin overexpression led to processing of only a small fraction of the total WT prM. In contrast, furin overexpression produced almost complete processing of prM H98A. Thus, we speculate that the prM H98A mutation may trap DENV in a conformational intermediate of the maturation pathway, and provide a tool to study this dynamic process. A number of other important questions on DENV particle conformation remain to be addressed. The packing of E dimers on the mature virus surface can be altered by exposure to the temperature range of the human body [51] , [52] . Although temperature does not affect the conformation of the fully immature virus [51] , it might affect processing intermediates such as that highlighted by prM H98A. Unlike DENV, low pH-triggered conversion to the furin-accessible form is irreversible for some flaviviruses [25] , perhaps due to differences in the interactions of prM H98. It is also possible that prM H98 plays additional roles within the typical ‘partially mature’ DENV, which would presumably contain some proportion of E proteins bound to the M region in the immature spike. Given the importance of DENV maturation in virus infectivity and antibody neutralization [28] , [53] , [54] , the maturation pathway is a fruitful area for future research. Cells and antibodies BHK-21, Vero and 293T cells were cultured in media at 37 °C [26] , [55] . 293T-furin cells that overexpress human furin were a gift from Dr Ted Pierson (NIAID) [42] . 4G2 is a mouse mAb recognizing the fusion loop of E protein of all flaviviruses including DENV [56] , [57] . DVB38.1 (here referred to as mAb 38.1) is a human mAb from a DENV3-infected patient and was a gift from Dr Aravinda M. de Silva (University of North Carolina). This antibody was shown to react with the prM protein by western blot [53] , and our western blot analysis showed that it recognized prM protein but not purified pr peptide or mature M protein, suggesting that the epitope is in the prM junction region. 4E11 is a mouse mAb that recognizes DIII of E protein of all DENV serotypes [58] , [59] , and was a gift from Dr Fernando Arenzana-Seisdedos (Institute Pasteur, Paris). Mouse polyclonal anti-DENV2 hyperimmune ascitic fluid was obtained from Dr Robert B. Tesh (University of Texas Medical Branch, Galveston). Western blot detection used mAb 4G2 for E protein, mAb 38.1 for prM (both used as 1:100 dilutions of a hybridoma culture supernatant), and a 1:10,000 dilution of a mAb to β-actin (Sigma) as a loading control. DENV1 prME expression and VLP The DENV1 virus-like particle (VLP) system was based on human codon-optimized prME from the DENV1 FGA/NA d1d strain (protein sequence 97.4% identical to WP strain) subcloned into a pcDNA expression vector, and was a gift from Dr Beatrice Nal (Hong Kong University-Pasteur Research Centre, Hong Kong) [39] . For prME processing and VLP secretion studies, 293T cells were transfected with the prME plasmid using calcium phosphate. Mature VLPs were produced by co-transfection of a furin-expressing plasmid (a gift from Dr Ted Pierson), and immature VLPs were produced by addition of 20 mM NH 4 Cl 12 h after transfection. For radiolabelling, the cells were incubated in Met- and Cys-deficient DMEM containing 35 S-Met and 35 S-Cys for 36 h starting at 12 h post transfection. To harvest, cell debris was removed from the culture medium by centrifugation at 10,000 r.p.m. in a Sorvall SS-34 rotor (12,000 g ) for 15 min. VLPs in the supernatant were pelleted through a 5% sucrose cushion by centrifugation in an SW41 rotor at 40,000 r.p.m. (273,000 g ) for 3 h. The pellet and cell lysate samples were analysed by SDS–PAGE and phosphorimaging, and prM processing was quantitated by determining the ratio of prM/(M+prM) using ImageJ and correcting for the number of Met/Cys in each protein. Western blot analysis was also performed where indicated to quantitate expression and secretion efficiency. For co-immunoprecipitation (co-IP) analyses, 293T cells were transfected with the prME plasmid and solubilized after 48 h in a lysis buffer containing either 50 mM Tris pH 7.4 or 50 mM MES pH 6.0, plus 150 mM NaCl, 1% NP40, 0.1% SDS and a protease inhibitor cocktail. After incubation for 1 h on ice, the lysates were cleared by centrifugation for 15 min at 12,000 r.p.m. (13,000 g ) in an Eppendorf microfuge. Five hundred micrograms (protein) of the cell lysate was then incubated overnight at 4 °C with 1.25 μg of mAb 38.1 against prM, or mAb 4E11 against E, plus 20 μl of protein G sepharose beads. The beads were washed with the corresponding lysis buffer, and viral proteins were detected by SDS–PAGE and western blot. DENV1 RVPs Constructs for the DENV1 western Pacific RVP system were a gift from Dr Ted Pierson [44] . For RVP production, 3 μg of the replicon plasmid pWNVII-Rep-GFPZeo and 12 μg of the pDV1-WP-structural protein plasmid encoding capsid-prM–E were transfected into 293T or 293T-furin cells using calcium phosphate. At 12 h post transfection, the medium was replaced with low-glucose DMEM plus 7% fetal calf serum (FCS) and the cells incubated at 29 °C for 36 h. RVPs in the medium were titered on Vero cells by scoring GFP-positive cells in the linear range. Radiolabelled RVPs were produced by incubation of the transfected 293T cells in Met- and Cys-deficient DMEM plus 35 S-Met and 35 S-Cys, 3% dialyzed FCS and 20 mM HEPES pH 7.0 at 29 °C for 36 h starting at 12 h post transfection. RVPs were concentrated by pelleting through a 20% sucrose cushion by centrifugation at 54,000 r.p.m. (249,000 g ) for 1 h using a TLS55 rotor, and then immunoprecipitated using mouse polyclonal anti-DENV2 serum. RVP secretion and processing were analysed and quantitated as described above for VLPs. DENV1 infectious clone, mutagenesis and revertants The DENV1 western Pacific infectious clone was a gift from Dr Barry Falgout [45] and used to generate the H98A mutant by site-directed mutagenesis [26] . Viral RNAs were transcribed and electroporated into 293T cells. Cultures were incubated 4 days in DMEM plus 2% FCS and 20 mM HEPES pH 7.0 at 29 °C. Progeny viruses were quantitated by infectious centre assay on indicator BHK-21 cells using mouse polyclonal anti-DENV2 serum [26] . Radiolabelled viruses were produced as detailed above for RVP, using culture for 4 days at 29 °C, and harvested and analysed as for RVP. To select for prM H98A revertants, 293T cells were electroporated with mutant viral RNA and cultured for 10 days at 29 °C. Virus in the culture media was then expanded by two passages for 5 days on naïve BHK-21 cells. Virus was pelleted, and the viral structural proteins sequenced by reverse transcriptase PCR [60] . Analysis of the positions of the revertants on the immature trimer structure was performed using PyMOL (The PyMOL Molecular Graphics System, Version 1.5.0.4 Schrödinger, LLC). Fusion infection assay Fusion of RVPs with the plasma membrane of BHK-21 cells was assayed as described for DENV [26] , [46] . Briefly, appropriate dilutions of mature DENV RVPs were prebound to BHK-21 cells for 90 min on ice in pH 8.0 binding buffer (RPMI without bicarbonate, plus 0.2%BSA, 10 mM HEPES and 20 mM NH 4 Cl), then treated at 37 °C for 1 min with medium buffered at the indicated pH to trigger RVP plasma membrane fusion. Cells were then cultured in complete BHK-21 medium containing 20 mM NH 4 Cl to prevent infection by the normal endocytic route. Twelve hours later, NH 4 Cl was removed and cells were cultured for another 36 h. Cells infected due to virus fusion were quantitated by GFP expression. How to cite this article : Zheng, A. et al. A toggle switch controls the low pH-triggered rearrangement and maturation of the dengue virus envelope proteins. Nat. Commun. 5:3877 doi: 10.1038/ncomms4877 (2014).